A haploid genetics toolbox forArabidopsis thaliana Genetic analysis in haploids provides unconventional yet powerful advantages not available in diploid organisms. In Arabidopsis thaliana, haploids can be generated through seeds by crossing a wild-type strain to a transgenic strain with altered centromeres. Here we report the development of an improved haploid inducer (HI) strain, SeedGFP-HI, that aids selection of haploid seeds prior to germination. We also show that haploids can be used as a tool to accelerate a variety of genetic analyses, specifically pyramiding multiple mutant combinations, forward mutagenesis screens, scaling down a tetraploid to lower ploidy levels and swapping of nuclear and cytoplasmic genomes. Furthermore, the A. thaliana HI can be used to produce haploids from a related species A. suecica and generate homozygous mutant plants from strong maternal gametophyte lethal alleles, which is not possible via conventional diploid genetics. Taken together, our results demonstrate the utility and power of haploid genetics in A. thaliana . Inbred (true-breeding) lines that are homozygous at virtually all loci enable both consistent production of superior hybrid plants as well as facile genetic analysis [1] , [2] , [3] , [4] . Traditional inbreeding, however, requires six to eight generations of selfing or sib-mating to generate inbred lines. For several crop species, haploid plants can be generated and subsequently doubled to produce true-breeding, entirely homozygous lines in two generations. Currently, the methods for haploid production vary depending on the species [1] , [2] . The most widely used method involves in vitro regeneration of plants from haploid cells or tissues, a procedure both tedious and expensive. Arabidopsis thaliana and many crop species have proven to be recalcitrant to in vitro haploid production [5] , [6] . In some species, wide crosses [7] , [8] , [9] , [10] , [11] , [12] or intraspecific crosses to lines with specific genetic determinants [13] , [14] result in in vivo haploid embryo because the chromosomes of the haploid inducer (HI) are lost during postzygotic mitotic divisions while the chromosomes of the non-inducer parent are retained [15] . In a majority of such species, the efficacy of in vivo haploid induction has been hindered by the need for tedious embryo rescue protocols that require in vitro cell culture. We have previously reported a breakthrough in in vivo haploid production: the generation of haploids through seed descent in A. thaliana by simple crossing of a wild-type (WT) strain to a transgenic strain expressing altered forms of CENH3, a centromere-specific histone [16] . Haploid production using altered CENH3 is particularly attractive and easy to adopt because viable haploid seeds are produced. Haploid genetics has long provided an invaluable tool for basic genetic research in both prokaryote and eukaryote microbial systems [17] , [18] , [19] and has recently been extended to mammalian systems through the generation of haploid cell lines [20] , [21] . However, although Arabidopsis remains a premiere model system for basic research in higher plants, haploid genetics has been largely inaccessible to the Arabidopsis research community. In this paper, we describe an improved version of the ‘green fluorescent protein (GFP)- tailswap ’ haploid induction method, demonstrating that haploid embryos are formed in association with chimeric endosperm and illustrate the utility of haploids in accelerating basic genetic analysis in A. thaliana . Our aim is to spur the utilization of haploid genetics across a wide array of genetic investigations and extend the potential of haploids as a genetic tool in plants. Specifically, we demonstrate that an A. thaliana HI can be used for the following: (1) swapping the cytoplasmic genome of one accession with the nuclear genome of another, (2) generating a series of lower euploids (3 × , 2 × , 1 × ) from a tetraploid (4 × ) parent, (3) rapid identification of recessive mutations in the M1 generation of a mutagenized population, (4) pyramiding of multiple mutant combinations and (5) generating plants that are homozygous for gametophyte lethal mutations. In addition, we also show that an A. thaliana HI line can be used to induce haploids from a sister species A. suecica through an interspecific cross, bypassing the need to develop an HI in the related species. Identification of haploid seed pre-germination Among our collection of variant CENH3 strains [16] , [22] , [23] , the previously described GFP- tailswap strain [16] is the optimal HI based on its haploid induction efficiency and ease of use (see Methods, Fig. 1a , Supplementary Fig. 1 ). The HI can be used either as a male or a female parent in a cross to generate maternal and paternal haploids, respectively [16] . This HI line produces 25–45% haploids when used as a maternal parent, whereas produces only 5% haploids if used as a paternal parent [16] . Furthermore, the HI parent produces few viable pollen [16] , [23] and thus we prefer to use HI as a female parent in crosses to produce haploids. F1 seed from HI × WT crosses produce a mixture of hybrid diploids, aneuploids and haploids in addition to a high frequency of aborted seeds [16] , [24] . 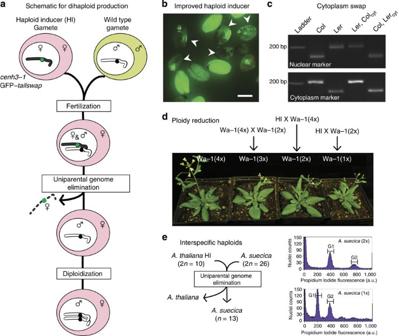Figure 1: Haploid toolbox forArabidopsis—Part I. (a) Cartoon of a (HI) cross depicting uniparental genome elimination. Any genotype of interest can be crossed as a male parent to the HI to induce haploid progeny. A green dot represents weak centromeres from the HI parent, while the black dot represents wild-type centromeres. The HI genome is eliminated after fertilization, producing seeds containing a haploid embryo. Note that haploids inherit the cytoplasm (coloured pink) from the HI parent. (b) SeedGFP-HI crosses produce two types of seeds: seeds with uniform GFP signal that develop as diploids or aneuploids and viable seeds showing mottled GFP fluorescence (arrow heads) which predominantly give rise to haploid progeny. Scale bar, 500 μm. (c) Gel electrophoresis image of PCR assays depicting cytoplasm transfer in haploids after a HI cross. Diploid WT Col-0 (lane 2) and Ler(lane 3) serves as controls for nuclear (top panel) and cytoplasmic (bottom panel) markers to show swapped cytoplasm in the haploids. A Lerhaploid in Col-0 cytoplasm (lane 4) and a Col-0 haploid in Lercytoplasm (lane 5) are shown here. (d) Images of 4 × , 3 × , 2 × and 1 × Wa-1 plant ploidy series are shown with the crossing scheme used for obtaining each of the above plants. (e) Diagram depicting an interspecific uniparental genome elimination cross betweenA. thalianaHI (2n=10) and the allotetraploidA. suecica(2n=26). Flow cytometric confirmation of ploidy reduction,A. suecicahaploid (2n=13) with half the nuclear content (bottom panel) compared with aA. suecicadiploid control (top panel). a.u., arbitrary units. Figure 1: Haploid toolbox for Arabidopsis —Part I. ( a ) Cartoon of a (HI) cross depicting uniparental genome elimination. Any genotype of interest can be crossed as a male parent to the HI to induce haploid progeny. A green dot represents weak centromeres from the HI parent, while the black dot represents wild-type centromeres. The HI genome is eliminated after fertilization, producing seeds containing a haploid embryo. Note that haploids inherit the cytoplasm (coloured pink) from the HI parent. ( b ) SeedGFP-HI crosses produce two types of seeds: seeds with uniform GFP signal that develop as diploids or aneuploids and viable seeds showing mottled GFP fluorescence (arrow heads) which predominantly give rise to haploid progeny. Scale bar, 500 μm. ( c ) Gel electrophoresis image of PCR assays depicting cytoplasm transfer in haploids after a HI cross. Diploid WT Col-0 (lane 2) and L er (lane 3) serves as controls for nuclear (top panel) and cytoplasmic (bottom panel) markers to show swapped cytoplasm in the haploids. A L er haploid in Col-0 cytoplasm (lane 4) and a Col-0 haploid in L er cytoplasm (lane 5) are shown here. ( d ) Images of 4 × , 3 × , 2 × and 1 × Wa-1 plant ploidy series are shown with the crossing scheme used for obtaining each of the above plants. ( e ) Diagram depicting an interspecific uniparental genome elimination cross between A. thaliana HI (2 n= 10) and the allotetraploid A. suecica (2 n= 26). Flow cytometric confirmation of ploidy reduction, A. suecica haploid (2 n= 13) with half the nuclear content (bottom panel) compared with a A. suecica diploid control (top panel). a.u., arbitrary units. Full size image The current HI requires all the F1 progeny to be grown to identify haploids demanding more growth space and time. Haploids can be identified by phenotypic, genotypic and cytological methods [16] , [24] (see Methods, Supplementary Fig. 2 ). A HI that allows the immediate identification of haploid seeds post harvest would allow selective planting of haploid progeny. For example, in Maize, haploid seeds can be selected using R1- nj anthocyanin marker system where hybrid diploid seeds show purple colour in both scutellum (embryo) and aleurone (endosperm) tissues, whereas haploid seeds display purple colouration only in the endosperm and not in the embryo [25] . Recently, an improved method based on oil content of haploid seeds has also been demonstrated for selection of maize haploids seeds [26] . To facilitate selection of haploid seeds in Arabidopsis crosses, we introduced the GFP fluorescent marker, expressed under the control of the seed storage protein 2S3 promoter ( At2S3: GFP) [27] into the HI strain, and named the resulting strain ‘SeedGFP-HI’. GFP signal in SeedGFP-HI is visible during late embryo development and persists in the embryo and endosperm [27] . We expected the diploid and aneuploid F1 seeds from a SeedGFP-HI cross to retain GFP fluorescence and haploid seeds to lack any signal in the embryo and endosperm. Examination of well-developed F1 seeds failed to identify seeds completely devoid of fluorescence ( Supplementary Fig. 3 ). Instead, we observed a mixture of uniformly fluorescent and mottled GFP fluorescent seeds ( Fig. 1b and Supplementary Fig. 3b and c ). In mottled GFP seeds, the GFP fluorescence was restricted to the endosperm and the embryo was devoid of GFP signal ( Supplementary Fig. 3d–j ). Next, we scored for GFP fluorescence in 3–5-day-old seedlings germinated from seeds that were either uniformly fluorescent ( n =50) or mottled ( n =193). All the seedlings from the uniformly fluorescent seeds ( Supplementary Fig. 3k,n ) showed GFP signal throughout the seedling ( Supplementary Fig. 3o,r ) and the resulting adult plants were hybrid diploids (16%), hybrid aneuploids (32%) and self-pollinated diploids (52%) ( Supplementary Table 1 ). In contrast, the mottled GFP seeds ( Supplementary Fig. 3l ) gave rise to seedlings devoid of GFP ( Supplementary Fig. 3p ), in agreement with our embryo dissection experiments ( Supplementary Fig. 3i,j ). When the seedlings were grown to maturity, 91% of these were haploids and the rest were aneuploids. These results indicate that pre-selection of mottled GFP seeds followed by selection of seedlings devoid of GFP signal increase the efficiency of early haploid selection. In addition, the association of haploid embryos to mottled endosperm poses the interesting question of how genome elimination is coordinated between zygotic tissues. Exchanging cytoplasmic and nuclear genomes In Arabidopsis , like in most crop species, the genomes of cytoplasmic organelles are inherited uniparentally from the mother via the egg cell. Despite the importance of maternal cytoplasm in breeding [28] , [29] , [30] , its effect on phenotype is not easy to ascertain because producing different nuclear versus cytoplasmic combinations normally requires hybridization followed by multiple generations of backcrossing. Genome elimination during haploid induction provides a rapid method for producing cytoplasm-swapped genotypes because the maternal cytoplasm is maintained while the entire maternal nuclear HI genome is eliminated [16] . For example, because HI originated from the Col-0 accession, all paternal haploids derived by crossing any accession to HI inherit the Col-0 cytoplasm ( Fig. 1c ). To demonstrate rapid and convenient swapping of cytoplasms, we generated a HI containing L er cytoplasm (see Methods) and pollinated this L er -cytoplasmic HI with Col-0 WT. Marker analysis confirmed that this cross generated Col-0 haploids with L er cytoplasm ( Fig. 1c ). This strategy can be employed to generate any desired combination of nuclear and cytoplasmic genome from the hundreds of natural accessions available for A. thaliana in only four generations ( Supplementary Fig. 4 ). Deconstructing a polyploid into a series of lesser euploids Deconstruction of a polyploid into a series of lower euploids can be achieved easily through HI. Autotetraploids have useful genetic characteristics because they exhibit increased tolerance to DNA damage and salt stress [31] . However, tetraploidy challenges genetic studies as a result of increased genetic redundancy and complicated tetrasomic inheritance [32] . We had previously shown that fertile Wa-1 diploids can be created by crossing the natural autotetraploid accession Wa-1 to HI (ref. 16 ). However, this diploid Wa-1 contains Col-0 cytoplasm inherited from maternal HI. Here we crossed the synthetic diploid Wa-1 as a pollen parent to natural tetraploid Wa-1 female to generate triploid Wa-1 plants containing Wa-1 cytoplasm. This triploid was subsequently crossed as a female to synthetic diploid Wa-1 male (Col-0 cytoplasm) to produce triploid, aneuploid and diploid progeny [33] , all with Wa-1 cytoplasm ( Supplementary Fig. 5 shows the crossing strategy to maintain Wa-1 cytoplasm in the ploidy series). Crossing the diploid Wa-1 subsequently to HI generated haploid Wa-1 ( Fig. 1d ). This full ploidy series can be used to study the effects of the different ploidy states in Arabidopsis . In addition, this strategy can be used to isolate mutant alleles from a polyploid background. Methods such as TILLING (Targeting Induced Local Lesions IN Genomes) can leverage the use a tetraploid population for mutagenesis because genetic redundancy allows for the recovery of greater mutation densities [34] . Further, dihaploid gametes should buffer against the lethal effects of severe alleles that are otherwise impossible to recover through haploid gametes. Thus, TILLING in a tetraploid increases the chance of finding a deleterious mutation in any gene of interest. However, a tetraploid TILLING plant carrying the desired mutant allele must be converted to diploid for easy genetic analysis. In fact, the cenh3-1 allele used to create the HI strain was originally isolated from a tetraploid TILLING population that conventionally required two transitional generations via a triploid bridge to generate a diploid CENH3/ cenh3-1 heterozygote [22] , [33] , [34] . With a HI strategy, we hypothesized that a tetraploid TILLING population can be converted to diploid by a single cross. To demonstrate this, we identified three new knock-out (KO) alleles (nonsense mutations) in SOG1 , a gene encoding a master regulator of DNA damage response [35] from the tetraploid TILLING population [34] and these heterozygotes were crossed onto HI diploid females. We recovered all three SOG1 KO alleles in the F1 progeny, from which five individuals were selected for further analysis. Flow cytometry on the selfed F2 progeny of these five lines confirmed the diploid nature of four progeny, one being aneuploid. Three putative diploids, each corresponding to a different sog1 KO allele, were further characterized via low coverage Illumina sequencing, and all three appeared to have balanced chromosome numbers as expected ( Supplementary Fig. 6 ). While generating mutants in a tetraploid has the disadvantage of adding one generation to the production of diploid mutants, this caveat is largely offset by the benefit of having to screen much smaller numbers of progeny, each carrying more mutations than individuals in diploid mutagenized populations [34] . Interspecific genome elimination Developing a HI strain in a new species demands time and effort. Therefore, it would be a significant advantage if a HI line could be used for uniparental genome elimination not only within its own species but also in crosses to closely related species. This is particularly relevant in a genus such as Brassica , where multiple commercially relevant crop species can be intercrossed to one another. We found that interspecific genome elimination is possible with our HI strategy. As a proof of concept, we crossed the allopolyploid species A. suecica (2 × =26) as a pollen parent with the A. thaliana GFP -tailswap HI strain (2 × =10). Out of 241 viable progeny, two were identified as A. suecica (2 × =13) based on their morphology and sterile phenotype. This was confirmed by flow cytometry and chromosome dosage analysis [36] ( Fig. 1e and Supplementary Fig. 7 ). Thus, an HI strain developed in one species can be successfully employed to generate haploids in a closely related species via interspecific crosses. The pitfalls to this approach are low recovery of hybrid seeds due to interspecies barrier, differences in parental chromosome numbers and endosperm imbalance. Despite these caveats, at least in the case of A. thaliana × A. suecica interspecific cross, this method appears to be straightforward and yields haploids with a frequency of at least 1%. Pyramiding of multiple mutant loci Plant breeding and classical genetics often require introgression of selected alleles at multiple loci. Following hybridization, a heterozygous F1 is selfed and the F2 population is screened for the desired homozygous genotype. The cost and complexity of this task increases exponentially with the number of loci according to the expression 1/4 n , where n represents the number of loci. For example, two loci result in 1/16 double homozygotes. In a haploid generation, the same frequency is calculated as 1/2 n instead. For example, for five loci, this produces a 32 × advantage, and 1 out of 32 haploid progeny is expected to inherit all 5 loci, as opposed to 1/1024 in the selfed diploid progeny ( Fig. 2a ). As a proof-of-principle, we crossed a triple heterozygous recessive mutant ( YUC1/yuc1;YUC2/yuc2;YUC8/yuc8 ) harbouring two independent marker constructs, DR5– GFP and an egg cell EC:Ds Red marker, both in hemizygous condition ( DR5 –GFP/−; EC:Ds –Red/−) to HI to generate haploids. Here the five mutations are not independent because the three YUC genes are on the long arm of chromosome 4. In addition, the positions of the two other markers are unknown. We obtained 2 individuals homozygous for all 5 loci out of 113 haploids (1/56.5). This is lower than expected, even if we consider all five loci to be unlinked (1/32), perhaps because of lower viability of the quintuple mutant or the presence of two mutations on sister chromatids of the same chromosome (unphased mutations) that require a meiotic recombination event for transmission to the same gamete. This experiment suggests that obtaining the same quintuple mutant via traditional diploid crosses would have been challenging and the fact that we were able to obtain two such individuals in a modest screen demonstrates the power of haploid genetics to rapidly generate complex genotypes. 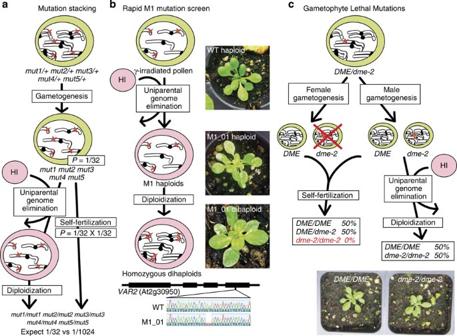Figure 2: Haploid toolbox forArabidopsis—Part II. (a) Cartoon comparing the generation of a quintuple mutant from a quintuple heterozygous parent by haploid genetics and conventional genetics. The haploid genetic scheme (left) has a 32 × advantage over the conventional diploid genetic scheme (right). (b) Schematic diagram showing the rapid recovery of phenotypic mutations in the M1 haploid generation using γ-irradiated pollen. Images of the M1_01 haploid mutant and its doubled haploid progeny with variegated leaf phenotype are shown. The candidate mutation that confers the M1_01 phenotype is a 2 bp deletion in exon 4 ofVAR2(At2g30950) but not in WT confirmed by Sanger sequencing as shown on the chromatogram. (c) Cartoon depicting the recovery of a homozygous female gametophyte lethal mutation.DME, a gene essential to the female gametophyte cannot be recovered through regular self-fertilization of diploid plants (left).dme-2male gametes fromDME/dme-2can successfully fertilize HI female gamete to give rise to haploiddme-2plants, which upon spontaneous chromosome doubling generate diploiddme-2/dme-2plants (right panel). Figure 2: Haploid toolbox for Arabidopsis —Part II. ( a ) Cartoon comparing the generation of a quintuple mutant from a quintuple heterozygous parent by haploid genetics and conventional genetics. The haploid genetic scheme (left) has a 32 × advantage over the conventional diploid genetic scheme (right). ( b ) Schematic diagram showing the rapid recovery of phenotypic mutations in the M1 haploid generation using γ-irradiated pollen. Images of the M1_01 haploid mutant and its doubled haploid progeny with variegated leaf phenotype are shown. The candidate mutation that confers the M1_01 phenotype is a 2 bp deletion in exon 4 of VAR2 (At2g30950) but not in WT confirmed by Sanger sequencing as shown on the chromatogram. ( c ) Cartoon depicting the recovery of a homozygous female gametophyte lethal mutation. DME , a gene essential to the female gametophyte cannot be recovered through regular self-fertilization of diploid plants (left). dme-2 male gametes from DME/dme-2 can successfully fertilize HI female gamete to give rise to haploid dme-2 plants, which upon spontaneous chromosome doubling generate diploid dme-2/dme-2 plants (right panel). Full size image Direct phenotypic characterization of recessive mutations Chemical mutagenesis and insertion element mutants are heterozygous in their first generation [34] , [37] and lesions of interest are often recessive and are therefore not visible in the phenotype of the mutagenized M1 population. Therefore, forward genetic screens require the production of M2 generations to allow recessive mutations to homozygose at the predicted 1/4 frequency. Functional genomics approaches such as forward and reverse genetic screens can be combined with haploid induction for faster analysis of non-lethal mutations. To demonstrate the principle of instantaneous screens, we combined mutagenesis of pollen followed by haploid induction to phenotypically screen for mutants in the M1 haploid generation. Specifically, pollen from L er gl1 plants was irradiated with varying doses of γ rays (100 Gy and 200 Gy) to induce double-stranded DNA breaks. The mutagenized pollen was used to pollinate the HI. Out of 240 haploids obtained (100 Gy irradiation), we obtained three phenotypically distinct haploid M1 mutants ( Supplementary Fig. 8 ). The M1_01 ( Fig. 2b ) mutant has mottled leaves, which phenocopies mutant phenotypes of VAR1, VAR2 and IMM . Analysis of mapped Illumina whole genome reads from M1_01 revealed a 2 bp indel in exon 4 of VAR2 (At2g30950) but not in L er gl1 haploid control. This lesion was further confirmed by targeted Sanger sequencing ( Fig. 2b ). This indel causes a frame shift, resulting in a non-functional truncated VAR2 protein that is a likely candidate for causing the variegated phenotype. We envision using haploid induction in this manner to significantly reduce the time and resources often associated with forward and reverse genetic screens. However, the disadvantage of using a haploid M1 screen is that mutations that need to be propagated in a heterozygous state, such as embryo lethal mutations and haploinsufficient gene mutations, cannot be obtained using this screen. Production of gametophyte lethal homozygous mutants Maternal and paternal gametophyte lethal mutations cannot be transmitted either through the female or male lineage, respectively [38] , [39] . It is therefore impossible to ascertain the loss-of-function phenotype of these genes on the sporophyte, except in the rare transmissions of weak alleles [38] . Because sex-specific lethal alleles can be transmitted through the unaffected sex, we hypothesize that haploid plants produced from the unaffected sex should inherit the mutant allele and permit the recovery of a mutant sporophyte. To test this hypothesis, we crossed maternal gametophytic lethal DME/dme-2 heterozygote [38] as the male to HI. Out of 37 haploids, we obtained 19 WT DME haploids and 18 dme-2 mutant haploids ( Supplementary Fig. 9 ). The 1:1 segregating ratio indicates that it is indeed possible to propagate maternal gametophyte lethal alleles as paternal haploid plants. The dme-2 mutant haploids were phenotypically similar to WT haploid siblings except for one sibling ( Supplementary Fig. 9 ), indicating that DME is not essential in adults. However, sporadic developmental abnormalities have been reported for homozygous mutant plants derived from heterozygous plants carrying the dme-1 weak allele, via transmission of the mutant allele through the female lineage [38] . These plants randomly produced individual flowers with reduced or increased floral organs mostly petals and sepals apart from improperly fused carpels, petaloid anthers, fused stamen filaments and so on [38] . In the case of the dme-1 weak allele, the abnormal floral phenotype was sporadically observed across random flowers in an inflorescence. When we produced haploid mutants carrying the dme-2 strong allele that show no female transmission, these abnormalities were confined to a single plant ( Supplementary Fig. 9b,c ) while all other mutant haploid plants ( n =17) looked WT ( Supplementary Fig. 9a ). Furthermore, floral abnormalities were observed almost uniformly across all the flowers in that single plant. This observation suggests that the developmental phenotype of this stronger allele of dme-2 is incompletely penetrant and manifests phenotypically only in certain mutant siblings. Similarly, mea-1 (ref. 39 ) haploids could also be obtained ( Supplementary Fig. 9 ). Surprisingly, both dme-2 and mea-1 haploids were partially fertile and produced diploid progeny that were homozygous recessive for their respective KO allele ( Fig. 2c ). The molecular basis for this unexpected result is currently being investigated. These results demonstrate the utility of this tool in determining the sporophytic phenotype of gametophyte lethal mutations and the importance of their characterization to understand gene function. We envision that the haploid genetic methods described in this study can in principle, be extended to any plant species for which a successful haploid production method exists. In vivo haploids are better suited for realizing the potential of haploids in basic genetics studies, especially in the case of methods such as swapping of nuclear and cytoplasmic genomes and for inducing interspecific uniparental genome elimination described here. Further, in a majority of crop species, in vitro production of haploids is genotype dependent [6] , [40] and cannot be exploited to its full advantage if multiple genotypes/strains are involved in the genetic experiments. Uniparental genome elimination leading to in vivo haploid production has been documented by plant breeders mostly from studies of interspecific hybridization experiments from several plant species [7] , [8] , [9] , [10] , [11] , [12] . In maize, an intraspecific in vivo haploid production system using Stock 6 genotype [13] derivatives is one of the commercially exploited haploid production system used for the development of hybrid maize cultivars [41] . However, the genetics behind both intraspecific and interspecific uniparental genome elimination are too poorly understood to engineer an in vivo haploid inducing system in any desired species. Recently, it has been shown in barley interspecific crosses ( Hordeum vulgare × H. bulbosum ) that elimination of H. bulbosum genome is associated with a selective loss of CENH3 from H. bulbosum centromeres, resulting in the production of haploids from H. vulgare [42] . This finding is encouraging because it links CENH3 function with genome elimination in an unrelated system. Engineering an in vivo haploid induction system through targeted manipulation of CENH3, as demonstrated in Arabidopsis [16] , could be successful in other plant species. A strategy for developing a CENH3-based haploid induction system in a plant species of interest are elaborated in a review [43] . Interestingly, a QTL mapping approach to identify the genetic loci behind haploid induction in Maize did not identify CENH3 loci, suggesting a different genetic mechanism in this case [44] . A better understanding of the maize uniparental genome elimination system and the CENH3-based haploid production system will pave a way towards employing in vivo -generated haploids for basic genetic studies besides their routine use for hybrid breeding in a wide variety of plant species. An insight that hints at the crucial role of the endosperm in haploid seed production came from our work with the seedGFP-HI strain and this should be considered as HI systems are developed in other species. The endosperm results from a double fertilization event and its development is sensitive to deviations from the 2:1 ratio of maternal/paternal genomes, as well as to specific epigenetic states of certain imprinted genes [45] . Haploid seed could be, in principle, associated with uniform triploid, uniform haploid or mottled endosperm. Failure of finding triploid endosperm–haploid embryo seed indicates coordination between the fates of HI chromosomes in the zygotes. Further, the absence of haploid endosperm–haploid embryo seed is most likely dependent on the necessity to maintain this ratio of parental genome dosage in the endosperm and implies that a failure to do so might underlie the large proportion of aborted seeds in an HI cross. We hypothesize that partial loss of mutant parent chromosomes in the endosperm might be responsible for the mottled GFP fluorescence seen in the endosperm of haploid seeds. This hypothesis is the subject of ongoing investigations. We have demonstrated novel facets of haploid genetics that will significantly reduce cost and time in comparison to currently employed approaches. In some cases, such as in the generation of homozygous recessives from sex-specific lethals, haploid induction has enabled the phenotypic characterization of a developmental stage that would otherwise be unattainable. Characterization of sex-lethal transmission after haploidization should add useful information on the function and regulation of these genes. These findings add to our previous work in which we demonstrated that haploids can be used to rapidly generate mapping populations [46] , chromosome substitution lines [47] , parental lines for reverse breeding [47] and for engineering clonal reproduction through seeds [48] . Finally, like in haploid yeast, it is possible to measure meiotic crossover and gene conversion using Arabidopsis haploids [49] and to study meiotic recombination events in the absence of a homologous partner during haploid meiosis [50] . Taken together, these methods constitute a novel and complementary genetic haploid toolbox for the Arabidopsis community. Plant materials and growth conditions Plants were grown in Sunshine Professional Peat-Lite Mix 4 (SunGro Horticulture) in a controlled environment growth room at 20°±3° with a 16 h/8 h light/dark photoperiod. The WT diploid (2 n =2 × =10) accessions used in this study are Col-0 and L er . DME/dme-2 and MEA/mea-1 plants are in L er background. The yuc1 (At4g32540) mutant is a SALK transfer DNA (SALK T-DNA) insertion mutant (Salk_106293) , yuc2 (At4g13260) mutant is Salk_030199 and the yuc8 (At4g28720) mutant is a dSpm insertion from the SLAT collection. L er gl1 pollen was used in M1 mutant screen for easy phenotypic identification of haploid plants. The tetraploid (2 n =4 × =20) Arabidopsis accession Wa-1 (CS6885) was obtained from the Arabidopsis Biological Resource Center (ABRC), Ohio State University. The tetraploid TILLING population used to identify the SOG1 lesion is of Col-0 accession and the seeds were obtained from UC Davis TILLING facility. A. suecica #1 (2 n =26), the allotetraploid used for the interspecific cross with A. thaliana HI was a strain described in the study by Hanfstingl et al. [51] Using and maintaining GFP -tailswap as a HI The HI used is homozygous for the cenh3-1 mutation as well as the GFP -tailswap transgene. GFP -tailswap/ GFP -tailswap cenh3-1/cenh3-1 plants (referred to as HI) that we have bred for haploid induction can be easily distinguished from WT plants by their bushy and stunted phenotype ( Supplementary Fig. 1a,b ). HI plants are predominantly male sterile during early to mid stages of the inflorescence growth, however, as the inflorescence matures distal flowers show increasing fertility and are more likely to self-pollinate. This is an advantageous feature for crossing and maintenance of HI genotype. First, male sterility in the early inflorescence allows pollination for haploid induction to be carried out without the need for tedious emasculation. Successful haploid induction has been achieved even in opened flowers (2–3 days after flower opening) as long as they have a receptive stigma. Even if accidental self-pollination occurs while crossing, the contaminant selfed progeny can be distinguished from haploids, hybrid diploids and aneuploids by the characteristic phenotype of HI plants as shown in Supplementary Fig. 1a . Second, viable seeds collected from self-pollinated siliques from later stages of inflorescence can be used to raise a uniform population of HI plants ( Supplementary Fig. 1b ), without the need to segregate out homozygous HI plants from a heterozygous parent. About 95% of such selfed seeds give rise to diploid HI plants that can be phenotypically distinguished from the 5% aneuploid siblings ( Supplementary Fig. 1b ). HI pistils elongate normally after successful pollination with viable pollen, which suggests that our HI has good female fertility. Because of the very low male fertility, self-pollination is minimal except in later stage flowers and thus unpollinated pistils fail to elongate. This property of HI can be used to distinguish a pollinated pistil from an unpollinated one while crossing. This is especially important when bulk pollen (collected by vacuum method) is randomly dusted onto open flowers. Even though siliques develop normally after successful crossing, about 70–95% of the developing seeds (depending on the Arabidopsis accession) within the silique abort during embryogenesis such that only 5–20% of viable seeds are typically recovered from a cross. Among the viable progeny, 40–60% are haploid with the remaining being either diploid or aneuploid. On an average, we recover ~1–3 haploid progeny per silique after crossing to a WT parent. Hence, we recommend crossing at least twice as many flowers as the required number of haploids. All HI lines used in these experiments were identified from a segregating population of a selfed CENH3/cenh3-1 GFP -tailswap/ GFP -tailswap individual by phenotype ( Supplementary Figs 1 and 2 ) and confirmed by PCR genotyping using a derived Cleaved Amplified Polymorphic Sequence (dCAPS) assay. Oligos used for genotyping are cenh3-1_XbaI_Fwd: 5′-AGAATTTTAGGTTTTTTATTTCGATTTTGTAACCCTAGATTTCGAATCTGAAATTTCTA-3′ and cenh3-1_XbaI_Rev: 5′-GCCTCTCCTTGTCGGGGTCTTCA-3′. The WT 212 bp CENH3 PCR product is cleaved by XbaI to produce a band at 148 bp but the mutant cenh3-1 allele remains uncut. Recovery of haploid and dihaploid progeny To maximize the recovery of haploid progeny from HI crosses, we recommend germinating F1 (HI × WT) seeds on MS (Murashige and Skoog) agar plates. We find that the late germinating seedlings (as late as 2–3 weeks after other siblings from the same cross) are enriched with haploid progeny. The chance of recovering the slowly germinating haploid progeny is maximized under the optimal conditions provided by MS agar. Haploid plants can be phenotypically distinguished from hybrid diploid, aneuploid and selfed siblings ( Supplementary Fig. 2a ) as early as 10 days post germination [16] . Yet another way to identify haploids is to screen for the presence of GFP fluorescence at centromeres by observing nuclei in different tissues ( Supplementary Fig. 2b,c ). Root tips from germinating seedlings can be used for early screening or flower parts such as petals, pistil or anthers can be used at later stages for scoring. Since haploids always originate from a parent devoid of centromeric GFP protein, plants without centromeric GFP protein are haploids. On the other hand, selfed HI progeny, hybrid diploid and aneuploid siblings display GFP fluorescence at their centromeres. Alternatively, haploid plants can be identified by PCR-based genotyping because they are homozygous for the WT CENH3 allele, whereas diploid and aneuploid siblings are heterozygous for the cenh3-1 allele contributed by the HI parent. In addition, the haploid plants can also be PCR tested for absence of the GFP -tailswap construct. For details on the primers and methodology for PCR-based genotyping, please refer to an earlier publication [24] . Final confirmation of haploids can be done by counting the number of chromosomes either in mitosis or meiosis ( Supplementary Fig. 2f,g ). For propagation and genetic analysis sterile haploids must be converted to fertile diploid plants called doubled haploids (DH). The traditional method to convert a haploid to a DH is to treat the plants with the microtubule depolymerizing drug colchicine. Although the latter works well, an eco-friendly way to produce DHs is to collect those spontaneous seeds from haploid plants produced as a result of spontaneous mitotic and/or meiotic chromosome doubling [16] . To achieve maximum harvest of spontaneous DH seeds, we recommend growing the haploid plants under optimal conditions, such as feeding with full strength MS nutrient solution, to achieve healthy growth. Under such conditions, the haploids tend to produce more flowers than WT diploid as a response to sterility. Production of more flowers increases the probability of spontaneous meiotic and/or mitotic doubling and the chances of obtaining DH seed. A single viable double haploid seed/plant is sufficient to propagate the genotype of that haploid plant. In practice, depending upon the accession, a single haploid typically produces 50 to 5,000 spontaneous DH seeds. Construction of seed marker HI line The binary vector pFP91 harbouring At2S3:: GFP [27] and introduced into Agrobacterium tumefaciens strain GV3101, which was used to transform a heterozygous CENH3/cenh3-1 GFP -tailswap/ GFP -tailswap plant by floral dip. Transformed GFP-positive T1 seeds harbouring At2S3:: GFP construct were identified by visualizing the seeds using a fluorescence stereomicroscope. GFP-positive seeds were selected and grown to identify CENH3/cenh3-1 GFP -tailswap/ GFP -tailswap T1 individuals. T2 seeds that show 100% inheritance of the At2S3:: GFP transgene were selected and selfed to ensured the stable expression of the endosperm marker in the T3 generation. A T3 plant of the genotype cenh3-1/cenh3-1 GFP -tailswap/ GFP -tailswap At2S3:: GFP /At2S3:: GFP was designated as ‘SeedGFP-HI’. The F1 seeds from SeedGFP-HI × Col-0 WT were broadly categorized into two groups based on the nature of GFP fluorescence:seeds with uniform GFP fluorescence and those with mottled GFP fluorescence ( Fig. 1b and Supplementary Fig. 3 ). Sorted seeds from each category were surface sterilized and sown on MS agar plates for germination. All plated seeds were labelled and imaged for GFP fluorescence using a fluorescence dissection stereomicroscope. After 3 days of cold treatment, the plates were transferred to the growth room. Germinating seedlings (3–5 days post germination) were imaged for GFP fluorescence and transferred to soil. The progeny were scored for ploidy as described above. Swapping of cytoplasm between L er and Col-0 accessions To generate the HI with L er cytoplasm ( Supplementary Fig. 4 ), a CENH3/cenh3-1 GFP -tailswap/ GFP -tailswap plant (Col-0) was used as a male parent and crossed to L er. Among the resulting F1, CENH3/cenh3-1 GFP -tailswap /− progeny was self-pollinated and the F2 segregant with cenh3-1/cenh3-1 GFP -tailswap with L er cytoplasm marked by characteristic phenotype of HI ( Supplementary Fig. 1a ) was crossed to Col-0 pollen. The resulting F1 seeds were germinated on soil and 30% ( n =56) of the established plants were phenotypically identified as haploid. To distinguish Col-0 and L er cytoplasm, a natural single nucleotide polymorphism in the chloroplast gene Atpt69346 was used in CAPS assay using the following oligos. CP717: 5′-GTCATTTACCCTGTTAGTCCG-3′ and CP718: 5′-GAAATACAAGACAGCCAATCC-3′. The PCR amplified product was then digested with the HinfI restriction enzyme and resolved on a 3.0% agarose gel ( Fig. 1c ). The nuclear genome of Col-0 and L er ecotype was differentiated using microsatellite marker nga8 located on chromosome 4. The microsatellite locus nga8 was PCR amplified using oligo combination CP662: 5′-TGGCTTTCGTTTATAAACATCC-3′ and CP663: 5′-GAGGGCAAATCTTTATTTCGG-3′ and the resulting products were resolved on a 3% agarose gel ( Fig. 1c ). Ploidy reduction of the Wa-1 tetraploid Ploidy reduction of the natural tetraploid Wa-1 was achieved by a two-step sequential genome elimination procedure as described above. A natural single nucleotide polymorphism between the Col-0 and Wa-1 chloroplast gene Atpt69346, which utilizes the same dCAPS assay [16] as described above was used to distinguish Col-0 and Wa-1 cytoplasm. The PCR amplified product is digested with the HinfI restriction enzyme, which cleaves the Wa-1 fragment twice and the Col-0 fragment once ( Supplementary Fig. 5 ). Diploidization of SOG1 mutation To identify new KO alleles for the SOG1 gene, we screened a TILLING population derived from 528 tetraploid ethyl methanesulfonate-mutagenized plants [34] . We identified three nonsense (KO) and 21 missense mutations in SOG1. Eight tetraploid plants representing each of the three sog1 KO alleles were genotyped by targeted Sanger sequencing of the SOG1 locus using following primers SOG_F1 5′-CTTTCACTGCTAGGTTGGGGT-3′, SOG_R1 5′-CTGTTGTGGCTGCTGGTAGA-3′ and SOGseq 5′-GATAATTCTGCTTTGTGTAG-3′. No plant was found to be homozygous for any of the three sog1 alleles. A heterozygous plant representing each mutation was crossed as pollen donor onto HI plants. Approximately 100 HI flowers were crossed for each line; the deposition of large quantities of pollen onto each flower was confirmed using a dissecting microscope. The HI plants were then bagged in a glycine bag to prevent contamination by diploids present in the same chamber. Viable seeds were rare (3–9 viable seeds/100 flowers crossed), reflecting the generally poor seed set obtained when crossing tetraploid Col-0 onto diploid Col-0 (ref. 45 ). The F1 seeds were sown on MS plates and the resulting seedlings were transplanted to soil and genotyped again by targeted Sanger sequencing. Plants carrying the mutation (heterozygotes) were identified and allowed to self-pollinate. To determine the frequency of diploids produced from HI × Tetraploid TILLING mutant crosses, ploidy analysis was done by flow cytometry on a bulk sample of 50 F2 seeds collected from each of the 5 F1 plants. Generation of A. suecica haploids To produce A. suecica haploids, interspecific crosses were performed by pollinating A. thaliana HI (2 n= 10) with pollen collected from A. suecica (2 n= 26) plants. The resulting F1 seeds were germinated on MS media and of the 576 germinated seedlings that were transplanted to the soil media only 241 survived. Only a small fraction of the 241 plants appeared to be phenotypically interspecific hybrids while the majority (~160) of the plants resulted from self-pollination of the HI. Flow cytometry and chromosome dosage analysis [36] using Illumina sequencing ( Supplementary Fig. 7 ) were used to confirm the haploid karyotype of the two A. suecica (2 n= × =13) plants. Multiple mutant analysis The YUC1/yuc1; YUC2/yuc2; YUC8/yuc8 triple heterozygous plants harbouring independent insertions of the DR5– GFP and EC::Ds RED transgene were genotyped by locus-specific PCRs detailed below. The haploids obtained after crossing this quintuple hetero/hemizygous mutant to the HI were PCR genotyped to identify homozygotes at all loci using the following set of oligos: The genotype for YUC1 locus (At4g32540) was identified using 5′-CCTGAAGCCAAGTAGGCACGTT-3′ and 5′-CGTTCATGTGTTGCCAAGGGAGATAC-3′ for the WT allele, followed by 5′-CCTGAAGCCAAGTAGGCACGTT-3′ and 5′-GGCAATCAGCTGTTGCCCGTCTCACTGGTG-3′ for T-DNA insertion. The WT YUC2 locus (At4g13260) was identified using 5′-CGTCCAATACCTTGAGTCTTACGC-3′ and 5′-CTGCATACAATCCGCTTTCGC-3′ and the T-DNA insertion was identified using 5′-GGCAATCAGCTGTTGCCCGTCTCACTGGTG-3′ and 5′-CTGCATACAATCCGCTTTCGC-3′ oligo pairs. Similarly for YUC8 (At4g28720), the WT allele was identified using 5′-CTAGTGCTCAACCGTCACAAACCCC-3′ and 5′-AACGTTGATTTACCCATTACTTCCCTCGG-3′ while the T-DNA allele was identified using the 5′-TACGAATAAGAGCGTCCATTTTAGAGGA-3′ and 5′-GAACTGACGCTTCGTCGGGTAC-3′ oligo pairs. The presence of EC::Ds Red transgene was identified by PCR using CP1118: 5′-GTCATCACCGAGTTCATGCGCT-3′ and CP1119: 5′-ACGCCGATGAACTTCACCTTGTA-3′. Lastly, DR5:: GFP was identified using oligo combinations CP844: 5′-ACAACAGCCACAACGTCTATATC-3′ and CP845: 5′-GGTGTTCTGCTGGTAGTGGTC-3′. The genomic location of the T-DNAs encoding the fluorescent DsRed and GFP markers was not determined. Haploid mutant M1 screen Bulked pollen from L er gl1 was collected using the vacuum collection method and exposed to 0 Gy (no irradiation), 100 Gy and 200 Gy of γ irradiation at the Center For Health and the Environment Facility in UC Davis. Irradiated pollen from the different treatments was used to pollinate HI plants. We observed very poor seed set from siliques pollinated with 200 Gy irradiated pollen, suggesting that this dose might be lethal to the male gametophyte. These crosses were not analyzed further. The 100 Gy pollen gave good seed set and the typical mixture of haploid, diploid and aneuploid progeny was recovered ( Supplementary Fig. 8 ). M1 haploids were scored based on their trichome-less L er gl1 phenotype of the male parent. Out of 240 haploids obtained from the 100 Gy cross, we identified three L er gl1 haploids exhibiting visible morphological mutant phenotypes ( Supplementary Fig. 8 ). Spontaneously produced DH seeds were collected from these plants and the DH mutants were recovered ( Fig. 2b ). DNA from WT L er gl1 and M1_01 were purified using DNA Phytopure Kit (GE) and sequencing libraries were prepared using the standard NEB Next DNA Library Prep with NEXTFlex-96 Adapters from BIOO Scientific and sequenced on Illumina HiSeq 2000. After mapping the reads to the Col-0 TAIR10 reference genome, a 2 bp indel in exon four of VAR2 (At2g30950) was identified in M1_01. To confirm the indel polymorphism, we designed primers VAR2_Fwd: 5′-AGTTGATGAAACTGAGTGTTTGAGACTGT-3′ and VAR2_Rev: 5′-GCCAATAGTTTCTTTCTCGAGAAGCACT-3′, and PCR amplified the fragment from WT and M1_01 for Sanger resequencing. Generation of homozygotes from gametophyte lethal mutants To generate dme-2 (At1g02580) and mea-1 (At5g04560) haploid mutants, heterozygous DME/dme-2 and MEA/mea-1 plants were crossed as pollen parent to HI plants. The resulting F1 seeds were directly sown on soil and the haploids were identified as described. All the haploids were PCR genotyped to identify the DME WT allele using CP1261: 5′-AGTAACTGATGTGTCCAAACCAGCTCC-3′ and CP1262: 5′-CTGCATTGTAAAACCACCATGGGTT-3′ oligo combinations, whereas haploids were PCR genotyped to identify the dme-2 mutant allele using CP1262 and a left border-specific oligo LB: GACGTGAATGTAGACACGTC-3′. In the case of MEDEA , the WT allele was identified using oligo combinations 5′-GCGTAGCAGTTAGGTCTTGCTG-3′ and 5′-GTTTGACCCGTCAGGACTCTC-3′, and the mea-1 allele using 5′-GCGTAGCAGTTAGGTCTTGCTG-3′ and 5′-CGTTCCGTTTTCGTTTTTTACC-3′. How to cite this article: Ravi, M. et al. A haploid genetics toolbox for Arabidopsis thaliana . Nat. Commun. 5:5334 doi: 10.1038/ncomms6334 (2014).